Organic semiconductor density of states controls the energy level alignment at electrode interfaces Minimizing charge carrier injection barriers and extraction losses at interfaces between organic semiconductors and metallic electrodes is critical for optimizing the performance of organic (opto-) electronic devices. Here, we implement a detailed electrostatic model, capable of reproducing the alignment between the electrode Fermi energy and the transport states in the organic semiconductor both qualitatively and quantitatively. Covering the full phenomenological range of interfacial energy level alignment regimes within a single, consistent framework and continuously connecting the limiting cases described by previously proposed models allows us to resolve conflicting views in the literature. Our results highlight the density of states in the organic semiconductor as a key factor. Its shape and, in particular, the energy distribution of electronic states tailing into the fundamental gap is found to determine both the minimum value of practically achievable injection barriers as well as their spatial profile, ranging from abrupt interface dipoles to extended band-bending regions. Organic electronics has tremendous potential for extending and complementing the range of conventional semiconductor applications and has, to some extent, already entered the market. This is especially true for organic light-emitting diodes (OLEDs) [1] , [2] , [3] , [4] , [5] , [6] in displays of mobile devices and, very recently, in television panels. In the fields of solid state lighting, integrated circuits based on organic field-effect transistors (OFETs) [7] , [8] , [9] , [10] , [11] and organic photovoltaic cells (OPVCs) [12] , [13] , [14] , [15] , [16] , commercial breakthrough is still ahead, with considerable effort in fundamental as well as applied research currently undertaken. All these devices have in common one or more organic semiconductor layer(s), possessing (as every semiconductor) a non-vanishing energy gap between occupied and empty electronic states. Electrical connection of the organic semiconductor(s) to peripheral circuitry, however, must inevitably be realized by metallic contacts, with a wide range of elemental metals and degenerately doped inorganic or organic semiconductors employed today [3] , [16] , [17] . These are characterized by a continuum of electronic states filled up to a common electron chemical potential, often referred to as the Fermi level, E F . Depending on the intended function of the organic electronic device, charges must either be injected from the metallic electrode into the organic semiconductor (OLED/OFET) or they must be collected from the organic semiconductor by the metallic electrode (OPVC) [18] , [19] . In Fig. 1a , a typical situation for the energetic alignment of all relevant electronic states is sketched schematically. We immediately realize that, in such a situation, charge carriers encounter energy barriers, Δ e for electrons and Δ h for holes, if they are to be injected and that, for their extraction, corresponding energy losses occur. This has led the community to acknowledge that minimizing these barriers/losses and, in a broader sense, controlling interfacial energy level alignment in general, is a key factor for improving device performance [18] , [20] , [21] , [22] , [23] , [24] , [25] , [26] , [27] , [28] , [29] . 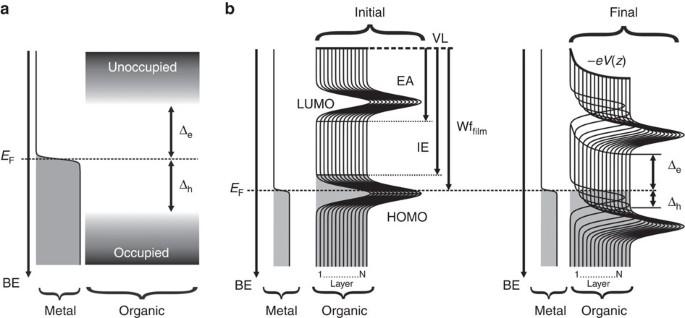Figure 1: Sketch of the energy level alignment at organic/electrode interfaces. (a) Schematic showing the Fermi-Dirac occupation function with Fermi levelEFfor the metallic side of the interface. The difference in binding energy (BE) betweenEFand the onsets of occupied and unoccupied density of states (DOS) on the organic semiconductor side are the charge injection barriers, Δhfor holes and Δefor electrons, respectively. (b) Example of a possible initial situation for the iterative electrostatic model described in the text. The energy differences between the onsets of the DOS derived from the highest occupied molecular orbitals (HOMOs) and the lowest unoccupied molecular orbitals (LUMOs) to the vacuum level (VL) define the ionization energy (IE) and the electron affinity (EA) of the organic semiconductor, respectively. The energy difference betweenEFand VL is the work function of the organic film (Wffilm). (c) Final energy level alignment after convergence of the iterative scheme discussed in the text. With increasing distancezfrom the electrode, the DOS increasingly shifts to higher BE by the local electron potential energy −eV(z), thus increasing Δhand decreasing Δewith respect to the initial situation. Figure 1: Sketch of the energy level alignment at organic/electrode interfaces. ( a ) Schematic showing the Fermi-Dirac occupation function with Fermi level E F for the metallic side of the interface. The difference in binding energy (BE) between E F and the onsets of occupied and unoccupied density of states (DOS) on the organic semiconductor side are the charge injection barriers, Δ h for holes and Δ e for electrons, respectively. ( b ) Example of a possible initial situation for the iterative electrostatic model described in the text. The energy differences between the onsets of the DOS derived from the highest occupied molecular orbitals (HOMOs) and the lowest unoccupied molecular orbitals (LUMOs) to the vacuum level (VL) define the ionization energy (IE) and the electron affinity (EA) of the organic semiconductor, respectively. The energy difference between E F and VL is the work function of the organic film (Wf film ). ( c ) Final energy level alignment after convergence of the iterative scheme discussed in the text. With increasing distance z from the electrode, the DOS increasingly shifts to higher BE by the local electron potential energy − eV ( z ), thus increasing Δ h and decreasing Δ e with respect to the initial situation. Full size image If, for a specific material pair, the situation sketched in Fig. 1a is found unsatisfactory, the obvious strategy is to reduce barriers/losses by either moving E F towards the occupied or unoccupied molecular levels (for example, by modifying the electrode work function or by choosing a different electrode material) or to move one of the molecular levels closer to E F (typically by choosing a different organic semiconductor). As the ultimate limit of such a strategy, one could assume that it was possible to eliminate barriers/losses altogether ( Fig. 1b ). In practice, however, this was only observed for monolayers of select molecules [30] , [31] , [32] , [33] , [34] , but could never be achieved for multilayer organic semiconductor films of device-relevant thickness. There, in contrast, non-vanishing energy barriers were found to remain ( Fig. 1c ). Several models have been developed in the past to explain this phenomenon [20] , [21] , [22] , [23] , [24] , [25] , [26] , [27] , [28] , [29] , [35] , [36] , [37] , [38] , [39] , [40] , [41] , each of which will be discussed to some detail in corresponding sections below. They differ not only in their intended range of applicability (from a single organic semiconductor layer [26] to thick films [23] , [25] , [27] , [29] ) but also in the envisioned regimes of electronic coupling strength between organic and electrode (from weak coupling with a passivated electrode [23] , [25] , [27] , [29] to intermediate coupling with an atomically clean metal [26] ) as well as in the assumed energy distribution of the electronic states in the organic (from discrete [23] , [25] , [29] to continuous [26] , [27] ). Here, we present results from a numerical electrostatic model, which allows treating all these various scenarios on equal footing. The full wealth of all encountered interfacial phenomena is described qualitatively and, provided required input data are available, even quantitatively [24] . With previous models naturally emerging as different limiting cases, we consolidate diverging views in literature regarding the physical origin of non-vanishing injection barriers (Fermi level pinning by metal-induced density of gap states [26] versus finite-temperature occupation of discrete molecular levels [23] , [25] ) as well as their spatial profile (interface dipole [26] , [29] versus band bending [25] , [27] ), and we provide a single, coherent framework for understanding the energy level alignment at interfaces between metallic electrodes and organic semiconductors. Introducing the model Our model is inspired by the earlier work of Vasquez et al . [26] , [39] and, more recently, of Blakesley et al . [27] , [28] , as well as of Greiner et al . [23] and Ley et al . [25] Going beyond refs 23 , 25 , however, we take into account a continuous density of states (DOS) both for the occupied and the unoccupied levels in the organic semiconductor. For simplicity, we start with the common choice [27] , [42] , [43] of one Gaussian peak, G ( E−E H , σ H ), arising from the energy distribution of the highest occupied molecular orbitals (HOMOs) and one, G ( E−E L , σ L ), from the distribution of the lowest unoccupied molecular orbitals (LUMOs) as indicated in Fig. 1b . To unambiguously define these peaks, both the energies of their maxima, E H and E L , and their standard deviations, σ H and σ L , need to be specified. The latter can be approximated, for example, by the width of the HOMO-derived feature observed in ultraviolet photoelectron spectroscopy (UPS). Here, we adapt the constant value of σ H = σ L =0.25 eV, found for the archetypical organic semiconductor pentacene [44] . From UPS and inverse photoelectron spectroscopy also the ionization energy (IE=4.8 eV) [44] and the electron affinity (EA=2.6 eV) [45] of pentacene are known. These quantities are typically determined from the energy difference between the vacuum level (VL) and the low-binding energy onset of the UPS spectrum and the high-binding energy onset of the inverse photoelectron spectroscopy spectrum, respectively. Choosing the onset of a Gaussian peak to be the energy, where the tangent through the inflection point crosses the base line, puts the peak centres 2 σ away from the so obtained onsets, that is, at E H =5.3 eV and E L =2.1 eV, respectively. Also indicated in Fig. 1b is the work function, Wf film , given by the energy difference between the Fermi level and the VL outside the organic semiconductor film. Note that, in the specific situation shown, Wf film is actually higher than the IE of the organic semiconductor, where electrons reside at energies above E F before charge equilibration. It is, therefore, clear that in the course of establishing a common electron chemical potential, charge will flow across the interface. To quantify the amount of transferred charge in the general case, we discretize the organic semiconductor film into layers of thickness Δ z and distance z from the electrode surface. We then calculate the charge density ρ ( z ) in each of these layers by integrating with e the (positive) elementary charge, n the number of molecules per unit area and per discretization interval Δ z . As the IE and EA values reported above pertain to pentacene molecules ‘standing’ on the electrode with their long molecular axes almost parallel to the surface normal [44] , [45] , we accordingly choose Δ z =1.42 nm, the distance d 001 between the crystallographic (001) planes in the pentacene single crystal [46] ; Δ z then corresponds to the height of one molecular layer. For the sake of simplicity, we consider layer-by-layer growth of pentacene only, with n =4.1 × 10 18 molecules/(m 2 ·Δ z ). Note, however, that fractional coverages and different growth modes could easily be incorporated by accordingly choosing layer-specific values for n . The first integral in the curly brackets of equation (1) yields the number of holes in the occupied DOS of the organic semiconductor and the second integral the number of electrons in the unoccupied DOS. While of noticeable consequence only for highly degenerate systems, we, nevertheless, follow refs 23 , 25 by allowing, in contrast to refs 27 , 28 , only single charging of each molecule, which slightly modifies the Fermi function for each individual energy level under consideration to Here, g H and g L are the HOMO and LUMO (spin-)degeneracies, both 2 in the case of pentacene, and β =1/ k B T with k B the Boltzmann constant and T the temperature, set to 300 K throughout the paper. Finally, the energy distributions of HOMO- and LUMO-derived levels are D H [ E+eV ( z )]= G [ E−E H + eV ( z ), σ H ] and D L [ E+eV ( z )]= G [ E−E L +eV ( z ), σ L ] in our model case, unless otherwise noted. We stress, however, that (i) any peak shape can be used instead of a Gaussian, (ii) each discretization interval could have a different DOS to account, for example, for image-charge screening by the metal, (iii) more molecular states can easily be taken into account by adding the respective terms in the curly brackets and (iv) potential temperature effects can be included in the standard deviation σ = σ(T) ; for the values used here, 2 σ =0.50 eV is about 20 times bigger than k B T at T =300 K and, therefore, the temperature dependence of f H/L ( E ) has only little impact on level alignment. Finally, the electrostatic potential across the organic semiconductor film, V ( z ), is first set to zero for calculating an initial guess of the charge density via equation (1). Once known, this ρ ( z ) serves to find the next V (z), which, going beyond refs 23 , 25 , we obtain by numerically solving the generalized one-dimensional Poisson equation with the discrete-difference method on a variable grid, using the second-order, central-difference scheme with mixed Dirichlet [ V (0)=0] and von Neumann [ V′ ( d )=0] boundary conditions, where d is the total thickness of the considered organic film and ε 0 the vacuum permittivity. For our first illustrative case of a homogenous pentacene film, we assume a static dielectric constant ε of ~3.6, as recently determined by impedance measurements [47] ; note, however, that each discretization interval could, in principle, also be given a different dielectric constant. The DOS of each discretization interval is then shifted in energy by the respective −e V ( z ), as shown in Fig. 1c , and the next ρ ( z ) is again generated by occupying all states in the organic up to E F . This self-consistent process is iterated until the difference in charge density between cycles is less than one electron per layer and square meter and the final injection barriers are obtained as Δ e = E F −EA and Δ h =IE− E F . Some illustrative results To illustrate the results delivered by the method just described, we first consider 20 layers (~30 nm) of standing pentacene with E F set to lie right at the energy of the HOMO peak maximum. The self-consistent solution of the Poisson equation for this situation is depicted in Fig. 2a,b , showing the charge density and the electron potential energy, respectively. The charge density rapidly vanishes with increasing distance from the electrode surface and reaches almost zero at 5 nm. The corresponding potential energy, which locally shifts HOMO, LUMO and VL by the same amount (IE and EA remain constant), is characteristic for band bending—a term somewhat liberally borrowed from inorganic semiconductor physics despite the fundamental difference that, instead of actual bands there, a distribution of localized states is assumed here. Although this phenomenon has often been attributed to (impurity or intentional) doping [29] , [48] , [49] in the past, it has recently been argued to arise also in intrinsic organic semiconductors, both of the conjugated-polymer [27] and the small-molecule variety [24] , [25] . In trying to relate our results to experimental observations, it is important to recall that the work function measured by, for example, UPS or Kelvin probe only reveals the electron potential energy − eV ( z ⩾ d ) just outside the organic film (highlighted in Fig. 2b ). As pointed out in refs 50 , 51 , 52 , 53 , however, the sequence of − eV ( d ) values obtained by increasing the total thickness d of an organic film in a step-wise manner and probing the surface potential at each step does not, in fact, recover the electron potential energy profile − eV ( z ) within the organic film for any thickness ( Fig. 2c ). 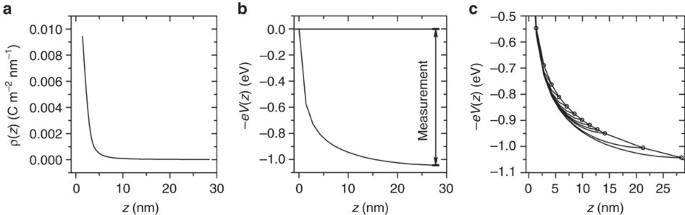Figure 2: Exemplary results of the iterative electrostatic model. (a) Calculated charge densityρ(z), and (b) electron potential energy −eV(z) within ad=30 nm thick (≈20 layer) pentacene film. Surface sensitive experimental methods (for example, UPS or Kelvin probe) only determine the total electron potential energy drop −eV(d) across the entire organic-semiconductor film. (c) −eV(z) for a range of different film thicknessesdup to 30 nm, highlighting that the series of experimentally determined −eV(d), shown as line connecting open circles, does not reproduce the band-bending −eV(z) within the organic semiconductor for any thickness. Figure 2: Exemplary results of the iterative electrostatic model. ( a ) Calculated charge density ρ (z), and ( b ) electron potential energy − eV ( z ) within a d =30 nm thick (≈20 layer) pentacene film. Surface sensitive experimental methods (for example, UPS or Kelvin probe) only determine the total electron potential energy drop − eV ( d ) across the entire organic-semiconductor film. ( c ) − eV ( z ) for a range of different film thicknesses d up to 30 nm, highlighting that the series of experimentally determined − eV ( d ), shown as line connecting open circles, does not reproduce the band-bending − eV ( z ) within the organic semiconductor for any thickness. Full size image Fermi level pinning With this in mind, we now plot in Fig. 3a the total potential energy change, − eV ( d ), across pentacene films of increasing d , for a series of different Fermi level energies. Clearly, when E F lies around mid-gap of the organic semiconductor, only very little charge is transferred from/to the metal electrode and, consequently, the potential energy profile remains close to flat. Upon E F approaching either the HOMO or the LUMO levels, however, pronounced charge transfer and, accordingly, ever higher and steeper potential energy changes across the organic film are obtained. Practically, the Fermi level is shifted by choosing electrodes of different work function, Wf elec , defined by the energy difference between E F and the VL just above the bare electrode surface with no organic material present. 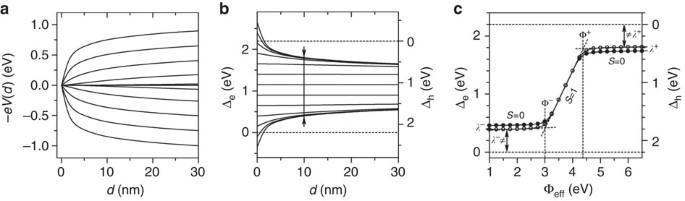Figure 3: Impact of effective substrate work function on band bending and barriers. (a) Total electron potential energy change −eV(d) across pentacene films of varying thicknessdfor a series of Fermi level energies ranging from 0.15 eV belowEL, the initial LUMO peak energy (top trace), to 0.05 eV aboveEH, the initial HOMO peak energy (bottom trace). (b) Data fromaconverted to injection barriers Δefor electrons (left axis) and Δhfor holes (right axis). Dashed horizontal lines indicate respective values of zero and the vertical line highlights the cut visualized inc. (c) Injection barriers Δe(left axis) and Δh(right axis) as a function of effective substrate work function Φefffor ad=10 nm thick pentacene film with (·) and without (○) polaronic relaxation energiesλ+(for holes) andλ−(for electrons) taken into account. The transitions between the regions with slopeS=0 andS=1 mark the so-called pinning work functions, Φ−for LUMO pinning and Φ+for HOMO pinning. The lowest achievable injection barriers are not related toλ+/−. The energy barriers/losses for charge carriers, Δ e and Δ h , are then related to Wf elec and − eV ( d ) through Figure 3: Impact of effective substrate work function on band bending and barriers. ( a ) Total electron potential energy change − eV ( d ) across pentacene films of varying thickness d for a series of Fermi level energies ranging from 0.15 eV below E L , the initial LUMO peak energy (top trace), to 0.05 eV above E H , the initial HOMO peak energy (bottom trace). ( b ) Data from a converted to injection barriers Δ e for electrons (left axis) and Δ h for holes (right axis). Dashed horizontal lines indicate respective values of zero and the vertical line highlights the cut visualized in c . ( c ) Injection barriers Δ e (left axis) and Δ h (right axis) as a function of effective substrate work function Φ eff for a d =10 nm thick pentacene film with (·) and without ( ○ ) polaronic relaxation energies λ + (for holes) and λ − (for electrons) taken into account. The transitions between the regions with slope S =0 and S =1 mark the so-called pinning work functions, Φ − for LUMO pinning and Φ + for HOMO pinning. The lowest achievable injection barriers are not related to λ +/− . Full size image where ID is the interface dipole. Either because of contamination through atmospheric and/or solvent exposure or owing to deliberate passivation with inert buffer layers, the ID is often found to be (close to) zero for practically employed electrodes in organic electronics. However, microscopic charge rearrangements originating in a variety of physical and/or chemical phenomena occurring between the electrode surface and the first organic layer can, in general, lead to appreciable IDs [22] , [37] , [38] , [54] , [55] , [56] . If available, for example, through a fully atomistic and quantum-mechanical treatment on a particular system, then they can, of course, be readily incorporated into the present model through equations (4) and (5). To study the impact of Wf elec on Δ e/h on more general grounds, however, we refer to an effective electrode work function in the following. Before charge equilibration, that is, with V ( d )=0, the initial barriers are then simply given by Δ e =Φ eff −EA and Δ h =IE−Φ eff , respectively. This now allows us to make the transition from relative potential energy changes for different values of E F ( Fig. 3a ) to absolute values of Δ e and Δ h for a series of effective electrode work functions, both of which are now quantities readily accessible through experiment. Figure 3b illustrates that changing Φ eff indeed permits tuning the interfacial energy barriers/losses, but only within a certain range. For our model case of pentacene, the achievable minimum separation between E F and EA/IE rapidly converges to Δ e =Δ h =0.4 eV with increasing film thickness, where decreasing Φ eff below ~3.0 eV does not further reduce Δ e and increasing Φ eff beyond ~4.4 eV does not further reduce Δ h . A more convenient way of visualizing these data is to directly plot the energy barriers as a function of Φ eff for a given film thickness, for example, d =10 nm as indicated by the vertical line in Fig. 3b . The obtained functional dependence (open symbols in Fig. 3c ) is characterized by a slope of zero ( S =0) for low Φ eff , a region with S =1 for intermediate Φ eff , and again S =0 for high Φ eff . The transitions between the different regions are marked by the so-called pinning work functions, Φ − =3.0 eV for LUMO and Φ + =4.4 eV for HOMO pinning with the latter matching the experimental value for a 10-nm film of pentacene [36] . The term pinning refers to the observation that, for multilayer organic semiconductor films of device-relevant thickness, E F cannot cross the HOMO or LUMO level onsets (marked as horizontal lines) and, thus, energy barriers/losses cannot be completely eliminated; regardless of the choice for Φ eff , the Fermi level appears to be ‘stuck’ at specific energy separations (~0.4 eV for d =10 nm) well above/below the respective peak onsets. In the past, this observation has led to the postulation of material-specific, discrete, quantum-mechanical states at these energies, the so-called ‘integer charge-transfer’ (ICT) states, with ICT + shifted up in energy from the HOMO onset and ICT − shifted down in energy from the LUMO onset into the gap of the organic semiconductor [29] . As already pointed out in refs 25 , 27 , 28 , however, the fact that the pinning energies of E F in the organic semiconductor gap emerge naturally (and quantitatively correct) from electrostatics alone: (i) lifts the necessity for invoking the existence of such states and (ii) invalidates the interpretation of their energy separation from the HOMO and LUMO onsets as the respective polaron-binding energies λ + and λ − . We explicitly illustrate this latter point in Fig. 3c for our Gaussian DOS ( cf. ref. 28 ). For our considered model case, pentacene, the polaron-binding energy, that is, the energy stabilization of an excess charge in the organic semiconductor by geometric relaxation of the charged molecule itself (internal relaxation energy) and of the surrounding lattice (external relaxation energy), was found to be only λ +/− =0.07 eV (refs 57 , 58 ) with the latter being negligible compared with the former [59] . This value is taken into account in equation (1) by shifting the HOMO and LUMO levels symmetrically towards each other, thus effectively reducing the gap of the organic semiconductor. The magnitude of the resulting changes (closed symbols in Fig. 3c ) is, not unexpectedly, comparable to the absolute value of λ +/− and, thus, its contribution to the observed minimum barriers is smaller than the typical experimental accuracy of ~0.1 eV; polaronic effects will, therefore, no longer be considered in the following. Film thickness and Gaussian DOS Briefly returning to Fig. 3b , it is evident that the relationship between Δ e/h and Φ eff changes with the total thickness of the organic film. In Fig. 4a , we show vertical cuts through the data presented in Fig. 3b not only for d =10 nm, as discussed in Fig. 3c , but for an entire series of thicknesses. As a direct consequence of band bending within the organic film, the substrate work functions where LUMO/HOMO pinning sets in successively decrease/increase with decreasing film thickness down to Φ − =~2.4 eV and Φ + =~4.7 eV, respectively, for a monolayer of pentacene, which, again, compares favourably to experiment [35] . Evidently, the thinner the organic semiconductor film, the lower Δ e and Δ h can be made by, respectively, decreasing or increasing Φ eff until, in the extreme case of a monolayer, they vanish for Φ eff =5.5 eV and Φ eff =1.8 eV, respectively ( cf. refs 30 , 31 , 32 , 33 ). 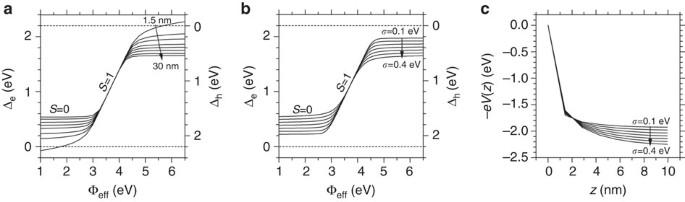Figure 4: Impact of film thickness and width of Gaussian DOS. (a) Injection barriers Δefor electrons (left axis) and Δhfor hole (right axis) as a function of effective substrate work function Φefffor pentacene films of thicknesses fromd=1.5 nm to 30 nm. (b) Injection barriers Δe(left axis) and Δh(right axis) as a function of Φefffor ad=10 nm thick pentacene film with the standard deviations of the Gaussian HOMO and LUMO DOS varied fromσH/L=0.1 eV up toσH/L=0.4 eV while retaining a constant IE and EA. (c) Electron potential energy profiles −eV(z) at the highest effective substrate work function Φeff=6.5 eV for allσH/Ltreated inb. Figure 4: Impact of film thickness and width of Gaussian DOS. ( a ) Injection barriers Δ e for electrons (left axis) and Δ h for hole (right axis) as a function of effective substrate work function Φ eff for pentacene films of thicknesses from d =1.5 nm to 30 nm. ( b ) Injection barriers Δ e (left axis) and Δ h (right axis) as a function of Φ eff for a d =10 nm thick pentacene film with the standard deviations of the Gaussian HOMO and LUMO DOS varied from σ H/L =0.1 eV up to σ H/L =0.4 eV while retaining a constant IE and EA. ( c ) Electron potential energy profiles − eV ( z ) at the highest effective substrate work function Φ eff =6.5 eV for all σ H/L treated in b . Full size image The same could, arguably, be achieved also for thicker layers if the DOS tailing into the gap of the organic could be eliminated; it is the presence and the occupation of these gap states, after all, that prevents E F from further approaching the HOMO/LUMO onsets. The origin of the gap states is commonly attributed to structural imperfection/defects [28] , [42] , [60] , [61] , [62] . Their density and energy distribution can experimentally be determined only on a case-by-case basis [60] , [61] , [62] , as they depend on specifics of sample preparation and environment, that is, exact film structure and composition [60] . To elucidate their impact on energy level alignment on more general grounds, we vary the width of the HOMO- and LUMO-related DOS while keeping it Gaussian-shaped, which has been shown to phenomenologically emulate also the impact of exponential tails [27] . Leaving, at the same time, the energies of the peak maxima, E H and E L , unchanged, trivially leads to the HOMO and LUMO onsets moving into the gap and, consequently, to E F getting pinned ever farther in the gap as well (not shown). A maybe less trivial result is presented in Fig. 4b . There, we keep the HOMO and LUMO onsets, which represent the physical material parameters IE and EA, respectively, at constant energy. Varying the width of the DOS then requires adjusting the energy separation between the peak maxima accordingly. Even under these conditions, however, reducing the Gaussian width of HOMO- and LUMO-related DOS leads to (i) the transition between the regimes of Fermi level pinning ( S =0) and the Schottky–Mott limit ( S =1) to become more abrupt, (ii) E F successively approaching the respective onsets in the pinning regimes and (iii) the spatial extent of the band-bending region to be reduced, as evidenced in Fig. 4c . The range of minimal energy barriers (~0.2 eV to ~0.6 eV) emerging from our model spans the entire range of values observed in experiment [44] , [55] , highlighting the decisive role of disorder in the organic semiconductor in determining interfacial energy level alignment [60] . Note also that, for T >0 K, finite barriers remain even in the limiting case σ H/L →0 of discrete molecular states, which is, in fact, the only case treated in refs 23 , 25 . From band bending to interface dipole Notably, the phenomenology described so far, the characteristic shape in Figs 3c and 4 in particular, is only ever observed for ‘weakly’ interacting electrode–organic interfaces. There, either through surface contamination or by design, the organic semiconductor is electronically decoupled from the metallic states by a thin, wide-gap buffer layer, which, in following refs 27 , 28 , we did not explicitly take into account so far. As shown in the Supplementary Discussion , even doing so does not alter the fact that the interfacial energy level alignment between organic semiconductor and metallic electrode always falls into one of three regimes, HOMO pinning, Schottky–Mott limit and LUMO pinning, characterized by slope parameters S =dΔ e /dΦ eff =−dΔ h /dΦ eff of (close to) zero, one and again zero, respectively (cf. Supplementary Figure 1 ). If, however, the buffer layer is eliminated completely in experiments, which can be achieved by, for example, depositing the organic semiconductor directly onto atomically clean metal surfaces in ultrahigh vacuum, also fractional slope parameters between 0 and 1 are frequently observed [26] , [36] , [39] , [55] , [63] . Despite having explored a good portion of the parameter space available in our model, we failed to generate non-integer values of S so far, whereas they are readily (and often quantitatively correct) predicted by the ‘induced density of interface states’ model [26] , [39] . This is surprising insofar, as this model is, in essence, quite similar to ours. Besides typically treating only molecular monolayers and assuming the organic DOS to be constant around E F for evaluating S , the main difference lies in the peak shape, which the authors take to be Lorentzian rather than Gaussian. This is entirely reasonable for the envisioned situation, where direct electronic coupling of the monolayer molecular levels to the metal leads to homogenous life-time broadening dominating over disorder-induced inhomogeneous (that is, Gaussian) broadening [60] . Having already elucidated the impact of the latter in Fig. 4b , we now choose a Voigt peak function with successively increasing Lorentzian weight to represent the DOS of the first organic layer, while retaining pure Gaussians for all subsequent layers. The Φ eff -dependence of the resulting injection barriers into a d =10 nm film of pentacene is shown in Fig. 5a , containing also the limiting, pure-Gaussian case already reported in Fig. 3c for comparison. 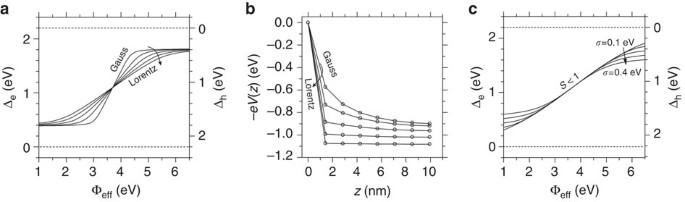Figure 5: Fractional slope parameters and band bending versus interface dipole. (a) Injection barriers Δefor electrons (left axis) and Δhfor hole (right axis) as a function of effective substrate work function Φefffor ad=10 nm pentacene film. The peak shape of the HOMO- and LUMO-derived DOS in the first layer is successively varied from pure Gaussian over Voigt to pure Lorentzian. (b) Electron potential energy −eV(z) within ad=10 nm pentacene film and a Φeffof 5.3 eV. Changing the peak shape of the HOMO- and LUMO-derived DOS in the first layer from pure Gaussian over Voigt to pure Lorentzian leads to a collapse of the spatially extended band-bending region to an interface dipole across the first molecular layer. (c) Injection barriers Δefor electrons (left axis) and Δhfor holes (right axis) as a function of effective substrate work function Φefffor ad=10 nm pentacene film. The DOS of the first layer is kept fixed to a Lorentzian peak shape of width 0.25 eV, whereas the standard deviationsσH/Lof the Gaussian peak shapes in all subsequent layers increase from 0.1 eV up to 0.4 eV. Although the range of linearity decreases succeedingly, the value of the slope parameter S<1 remains unchanged. Figure 5: Fractional slope parameters and band bending versus interface dipole. ( a ) Injection barriers Δ e for electrons (left axis) and Δ h for hole (right axis) as a function of effective substrate work function Φ eff for a d =10 nm pentacene film. The peak shape of the HOMO- and LUMO-derived DOS in the first layer is successively varied from pure Gaussian over Voigt to pure Lorentzian. ( b ) Electron potential energy − eV ( z ) within a d =10 nm pentacene film and a Φ eff of 5.3 eV. Changing the peak shape of the HOMO- and LUMO-derived DOS in the first layer from pure Gaussian over Voigt to pure Lorentzian leads to a collapse of the spatially extended band-bending region to an interface dipole across the first molecular layer. ( c ) Injection barriers Δ e for electrons (left axis) and Δ h for holes (right axis) as a function of effective substrate work function Φ eff for a d =10 nm pentacene film. The DOS of the first layer is kept fixed to a Lorentzian peak shape of width 0.25 eV, whereas the standard deviations σ H/L of the Gaussian peak shapes in all subsequent layers increase from 0.1 eV up to 0.4 eV. Although the range of linearity decreases succeedingly, the value of the slope parameter S<1 remains unchanged. Full size image Clearly, with increasing weight of the Lorentzian contribution, ever lower/higher substrate work functions are required to reach the same barriers for electrons/holes. More importantly, however, the Φ eff -region of non-vanishing slope parameter expands, where S itself decreases from unity to a value of 0.42 for a Lorentz dominated (75%), down to 0.35 for an exclusively Lorentzian DOS, which brackets the experimental observed values of 0.37 and 0.40 for pentacene [55] , [63] . This remarkable transition between phenomenologically distinct energy level alignment regimes is accompanied by profound changes in the electron potential energy profile − eV ( z ) within the organic semiconductor film ( Fig. 5b ). On increasing the Lorentz weight in the first-layer DOS, the spatially extended band-bending region in the organic is successively compressed towards the immediate interface with the electrode until, in the case of a pure Lorentzian, it collapses into a potential energy step across only the very first molecular layer. The abruptness of this step, which is not a unique feature of the Lorentzian peak shape per se but simply a consequence of the (compared to the Gaussian) higher DOS around E F , has led to it being assimilated into the interface dipole (as defined above) in the past. This can be justified by considering that the combined action of all interfacial effects reduces the work function that subsequently deposited molecules ‘see’ to, in our case, Φ eff −e V ( d )=6.5 eV−2.1 eV=4.4 eV, which is, again, the HOMO-pinning work function Φ + of pentacene. Therefore, no further charge transfer between the monolayer-covered electrode and succeeding organic semiconductor layers occurs and, with Δ h having reached its minimum value of 0.4 eV already, no additional shifts in electron potential energy arise. Deviation from a strictly linear evolution of Δ h/e is not observed until the Gaussian DOS of subsequent bulk layers again tails across E F for extreme values of Φ eff , thereby causing residual band bending. The range of linearity is thus restricted by the amount of energetic disorder in the bulk (exemplified by σ H/L -values ranging from 0.1 eV up to 0.4 eV in Fig. 5c ), but the absolute value of the slope parameter S<1 is not affected. This noteworthy result rationalizes the success of the induced density of interface state model in correctly reproducing the interfacial energy level alignment in the limiting case of atomically clean metals with intermediate work functions, despite it considering only monolayer coverage. To summarize, we present the results of a single, versatile electrostatic model, from which all observed regimes of energy level alignment at metal/(insulator/)organic semiconductor interfaces emerge naturally. Although designed to accommodate unprecedented detail and complexity, it contains prior work as limiting cases, notably, that of Ley et al . [25] , which is limited to producing either VL alignment ( S =1) or Fermi level pinning ( S =0) as a consequence of considering only discrete molecular states; that of Blakesley et al . [27] , [28] , which does not explicitly include insulating buffer layers and, thus, overestimates interfacial charge densities, as shown in the Supplementary Discussion ; and that of Vazquez et al . [26] , which is limited to a single molecular layer with Lorentzian DOS and, thus, fails to predict band bending. In providing a unified picture of the underlying physical mechanisms, our model confirms that the DOS of the organic semiconductor is the central, decisive quantity, responsible for all experimentally encountered phenomena and that controlling it is, therefore, key to minimizing charge carrier injection barriers and/or extraction losses beyond what is possible by adjusting the electrode work function alone. Using high (for holes) and low (for electrons) work-function electrodes is, of course, still a necessary prerequisite. Our results illustrate, however, that there are intrinsic limits to this strategy and that, to overcome these limits, the amount of electronic states in the energy gap of the organic semiconductor (as well as their energetic separation from its band edges) must be reduced. Besides eliminating defects within the organic semiconductor, our model suggests electronic decoupling from the metallic electrode to be a critical component in achieving this, thereby providing a theoretically well-founded justification for the wide-spread use of thin passivating buffer layers. As a further beneficial consequence of ‘cleaning out the gap’, spatially extended band-bending regions are predicted to develop within the organic semiconductor, which, in contrast to sharply localized interface dipoles, further lower effective injection barriers in OLEDs under applied bias voltage and facilitate the efficient collection of photo-generated charge carriers in OPVCs by imposing a drift direction. Our results thus provide a solid theoretical basis for past and present efforts in optimizing the interfacial energy level alignment at organic semiconductor/electrode contacts and will, hopefully, inspire future work. How to cite this article: Oehzelt, M. et al . Organic semiconductor density of states controls the energy level alignment at electrode interfaces. Nat. Commun. 5:4174 doi: 10.1038/ncomms5174 (2014).